Activity-dependent facilitation of Synaptojanin and synaptic vesicle recycling by the Minibrain kinase Phosphorylation has emerged as a crucial regulatory mechanism in the nervous system to integrate the dynamic signalling required for proper synaptic development, function and plasticity, particularly during changes in neuronal activity. Here we present evidence that Minibrain (Mnb; also known as Dyrk1A), a serine/threonine kinase implicated in autism spectrum disorder and Down syndrome, is required presynaptically for normal synaptic growth and rapid synaptic vesicle endocytosis at the Drosophila neuromuscular junction (NMJ). We find that Mnb-dependent phosphorylation of Synaptojanin (Synj) is required, in vivo , for complex endocytic protein interactions and to enhance Synj activity. Neuronal stimulation drives Mnb mobilization to endocytic zones and triggers Mnb-dependent phosphorylation of Synj. Our data identify Mnb as a synaptic kinase that promotes efficient synaptic vesicle recycling by dynamically calibrating Synj function at the Drosophila NMJ, and in turn endocytic capacity, to adapt to conditions of high synaptic activity. Coordinated phosphorylation and dephosphorylation of endocytic proteins located in the presynaptic terminals have been shown to dynamically regulate the efficacy of synaptic vesicle recycling and to ensure robust and reliable neurotransmission across a wide range of activity [1] , [2] , [3] , [4] , [5] . Yet, despite the identification of over 500 genes that encode kinase in the human genome [6] , our knowledge of the kinases that function at synapses, their targets and the mechanisms underlying their regulation of synaptic transmission in vivo remain limited. The Minibrain kinase (Mnb), also called the dual-specificity tyrosine kinase 1A (Dyrk1A), is a functionally diverse proline-directed serine/threonine kinase known to be mutated in autism spectrum disorder and upregulated in Down syndrome [7] , [8] , [9] , [10] , [11] . Mnb/Dyrk1A phosphorylates proteins with consensus target sequences RPX(S/T)P or RX(S/T)P [12] , [13] ; however, it has been particularly difficult to predict the in vivo substrates, as many of the proteins identified to date do not match the classical consensus sequences. Studies have shown that fly mnb mutants have smaller brains, reduced neuronal proliferation and locomotor defects [14] . Haploinsufficient Dyrk1A +/− mice also have smaller brains with fewer neurons and altered learning and memory performance [15] , [16] , whereas Dyrk1A/Mnb transgenic mice have learning and memory impairment as well as locomotor defects [17] , [18] . These results suggest that Dyrk1A/Mnb is particularly sensitive to dosage perturbations and has important roles in the nervous system, including neurogenesis, neuronal differentiation and learning and memory [15] , [17] , [19] , [20] , [21] , [22] . In neurons, Dyrk1A/Mnb is found in the nucleus and cytoplasm, as well as at the synapse [20] , [23] , [24] . Because of its putative role in neurogenesis and neuronal proliferation, much of the research has focused on the nuclear function of Dyrk1A/Mnb, given its ability to phosphorylate cyclin and other transcription and splicing factors [19] . However, the in vivo function of Dyrk1A/Mnb at the synapse, if any, remains unexplored. In vitro studies have shown that Dyrk1A/Mnb can phosphorylate multiple clathrin and endocytic- associated proteins, including Synaptojanin 1 (Synj) and dynamin [25] , [26] , [27] . However, the physiological significance of Dyrk1A/Mnb-mediated phosphorylation on synaptic function remains unknown. Synj is a phosphoinositol phosphatase that interacts with other endocytic proteins, including Endophilin (Endo) and Dap160/intersectin via its proline-rich domain (PRD) to facilitate synaptic vesicle endocytosis [28] , [29] , [30] , [31] , [32] , [33] , [34] . synj mutations in vertebrates and invertebrates lead to the accumulation of densely coated vesicles, suggesting that Synj functions in clathrin uncoating [30] , [31] , [35] , [36] . Studies have also demonstrated that Synj activity and interaction with Endo can be inhibited by kinases such as cyclin-dependent kinase 5 (Cdk5) and the ephrin receptor [37] , [38] , underscoring the possibility that Synj may undergo dynamic regulation to facilitate endocytosis. To investigate the synaptic functions of Dyrk1A/Mnb in vivo , we characterized the effects of mnb mutations at the Drosophila larval neuromuscular junction (NMJ). The fly NMJ is a glutamatergic synapse and an excellent model for studying genes and mechanisms regulating synaptic vesicle recycling, with many endocytic genes shown to have conserved functions in the vertebrate central nervous system [39] . Our results reveal that Mnb is a kinase that specifically enhances Synj phosphoinositol phosphatase activity to accelerate synaptic vesicle endocytosis during conditions of high activity. mnb mutants exhibit altered synaptic growth and morphology, as well as impaired synaptic vesicle endocytosis. Biochemical experiments reveal that Mnb phosphorylates Synj and alters endocytic protein interactions. Interestingly, overexpression of synj significantly rescued mnb phenotypes, consistent with Synj being a substrate of Mnb. Although it is known that the rate of synaptic vesicle endocytosis can be enhanced during periods of high activity to maintain a functional vesicle pool, neuronal signal transduction mechanisms that couple synaptic demand to efficient synaptic vesicle recycling is not well understood. Our findings that synaptic activity increases Mnb mobilization to endocytic zones and enhances synaptic Synj phosphorylation and activity further suggests that Mnb promotes efficient synaptic vesicle recycling by dynamically regulating Synj function during periods of robust synaptic activity. Mnb is enriched in the presynaptic terminals of the Drosophila NMJ To understand the role of Mnb in synaptic function, we first determined the localization of the Mnb protein by generating an antibody that recognizes all Mnb isoforms ( Fig. 1a and Supplementary Fig. 1a ). Western blot analyses revealed that Mnb is enriched in the Drosophila nervous system. Three main bands were detected at ~100, 69 and 66 kDa, close to the 96, 66 and 65 kDa predicted for Mnb-E, Mnb-F and Mnb-G, respectively ( Fig. 1b ). Mnb-H and Mnb-I, which have predicted molecular weight of 111.1 and 81.1 kDa, respectively, were below the level of detection. Specifically, Mnb-F and Mnb-G are enriched in the adult heads and larval brains, whereas Mnb-E is found in both the body muscle wall and the brain. This result is consistent with our quantitative reverse transcription PCR (RT–PCR) results, which showed that Mnb-F is the predominant isoform found in the nervous system ( Supplementary Fig. 1b ). 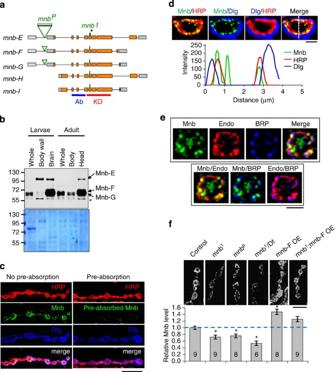Figure 1: Mnb is found in the presynaptic terminals ofDrosophilaneuromuscular junction. (a) Schema of predictedmnbisoforms. Orange boxes indicate translated region and grey boxes show untranslated mRNA. Green lines and inverse triangles indicate mutant alleles. *ATP binding site in the kinase domain (KD). Blue line indicates region used to generate MNB antibody (Ab). (b) Representative western blotting showing enrichment of Mnb isoforms in the larval brain and adult head extracts. ‘Whole’ indicates protein extracts prepared from the whole animal during either larval or adult stage. *A band at 60 kDa that does not correspond to the size of any known Mnb and hence is either a nonspecific signal or a currently unidentified Mnb isoform. Lower blot shows DB71 stained nitrocellulose membrane, indicating comparable amount of total protein (10 μg) loaded in each lane. (c) Third instar NMJ of muscle 6/7 at A2 immunostained by antibody that recognizes MNB or with antibody that had been pre-absorbed with purified immunizing Mnb protein. Mnb colocalizes with HRP but not Dlg, indicating the presence in the presynaptic terminal. Scale bar, 10 μm. (d) Image of a single bouton and the intensity plot profile for each antibody across the bouton (dotted white line). Mnb staining is confined within the boundaries of HRP staining, and is therefore presynaptic. Scale bar, 2 μm. (e) Image of a single bouton stained with Mnb, Endo and BRP to show colocalization of Mnb with subdomains of Endo in the periactive zone. Mnb did not colocalize with BRP. Scale bar, 2 μm. (f) Levels of Mnb staining within the NMJ of third instar larvae of the indicated genotype. Scale bar, 10 μm. Sample numbers are indicated in the graph. *P<0.05 compared with control. All values indicate mean±s.e.m. Figure 1: Mnb is found in the presynaptic terminals of Drosophila neuromuscular junction. ( a ) Schema of predicted mnb isoforms. Orange boxes indicate translated region and grey boxes show untranslated mRNA. Green lines and inverse triangles indicate mutant alleles. *ATP binding site in the kinase domain (KD). Blue line indicates region used to generate MNB antibody (Ab). ( b ) Representative western blotting showing enrichment of Mnb isoforms in the larval brain and adult head extracts. ‘Whole’ indicates protein extracts prepared from the whole animal during either larval or adult stage. *A band at 60 kDa that does not correspond to the size of any known Mnb and hence is either a nonspecific signal or a currently unidentified Mnb isoform. Lower blot shows DB71 stained nitrocellulose membrane, indicating comparable amount of total protein (10 μg) loaded in each lane. ( c ) Third instar NMJ of muscle 6/7 at A2 immunostained by antibody that recognizes MNB or with antibody that had been pre-absorbed with purified immunizing Mnb protein. Mnb colocalizes with HRP but not Dlg, indicating the presence in the presynaptic terminal. Scale bar, 10 μm. ( d ) Image of a single bouton and the intensity plot profile for each antibody across the bouton (dotted white line). Mnb staining is confined within the boundaries of HRP staining, and is therefore presynaptic. Scale bar, 2 μm. ( e ) Image of a single bouton stained with Mnb, Endo and BRP to show colocalization of Mnb with subdomains of Endo in the periactive zone. Mnb did not colocalize with BRP. Scale bar, 2 μm. ( f ) Levels of Mnb staining within the NMJ of third instar larvae of the indicated genotype. Scale bar, 10 μm. Sample numbers are indicated in the graph. * P <0.05 compared with control. All values indicate mean±s.e.m. Full size image We next used immunocytochemistry to determine whether Mnb protein is present at the NMJ. Figure 1c,d show that Mnb is enriched presynaptically within the boundaries of horseradish peroxidase (HRP) staining, a marker for the presynaptic membrane, and does not overlap with disc-large (Dlg), a postsynaptic maker. Immunostaining of the NMJ using Mnb antibody that had been preabsorbed with the immunizing protein ( Fig. 1c ) further confirms the specificity of Mnb staining and indicates Mnb is enriched in the presynaptic boutons of the Drosophila NMJ, consistent with a recent report that demonstrated Dyrk1A is found in a subset of motor neurons and present in the mouse NMJ [24] . To gain insights into the functional aspects of Mnb kinase in the synapse, we further defined Mnb distribution within the synaptic terminals. We observed partial colocalization of Mnb with either Endo or Dap160, endocytic proteins found in the periactive zone [33] , [34] , [40] ( Fig. 1e and Supplementary Fig. 1c ). Although punctate, Mnb did not colocalize with bruchpilot (BRP), an active zone marker. Together, these results indicate Mnb is enriched in periactive zones of the synapse, areas implicated in synaptic vesicle recycling. Mnb is required for synaptic growth Synaptic kinases have been shown to play a major role in sculpting the synapse by either promoting or restraining synaptic growth [41] , [42] . Previous studies in flies and mice have demonstrated that null mutations in mnb cause embryonic lethality [15] , [43] . To circumvent this limitation, we used hypomorphic alleles of mnb . mnb f0137 (referred to as mnb P ), a mutant with a transposon insertion in the 5′-untranslated region of the mnb gene ( Fig. 1a ), displayed a mild reduction in the level of overall Mnb protein as assessed by western blottings and specifically in the synapse as indicated by immunostaining ( Fig. 1f and Supplementary Fig. 1d ). mnb 1 , the classical mnb mutant, which harbours a point mutation next to the critical ATP binding residue in the kinase-active site previously shown to influence both Mnb function and protein level [14] , also showed a corresponding decrease in Mnb levels in the synaptic terminal. To further reduce Mnb protein levels, we generated mnb 1 alleles in trans to a mnb deficiency allele ( mnb 1 / Df ), which exhibited a ~10% survival rate and displayed the largest reduction in Mnb levels ( Fig. 1f and Supplementary Fig. 1d ). As the mnb-F isoform is the most abundant isoform found in neurons, we also generated transgenic flies expressing mnb-F using the UAS/GAL4 system. Figure 1f and Supplementary Fig. 1e show that expression of mnb-F using the pan-neuronal synaptobrevin-Gal4 driver ( nsyb-Gal4 ) indeed resulted in higher levels of Mnb. We examined synaptic morphology in different mnb alleles by immunostaining the NMJ with HRP. Reducing Mnb levels led to an undergrowth phenotype, with the NMJs showing a profound decrease in the number of synaptic boutons, but an increase in the size of these terminals ( Fig. 2 ). mnb 1 / Df showed the most striking changes in synaptic morphology. Interestingly, presynaptic overexpression of mnb-F resulted in the opposite phenotype, namely an increase in the number of smaller boutons ( Fig. 2 ). Overexpression of mnb-F in neurons of mnb 1 mutant restored the number and size of synaptic boutons back to normal, demonstrating that Mnb functions presynaptically to control synaptic growth. 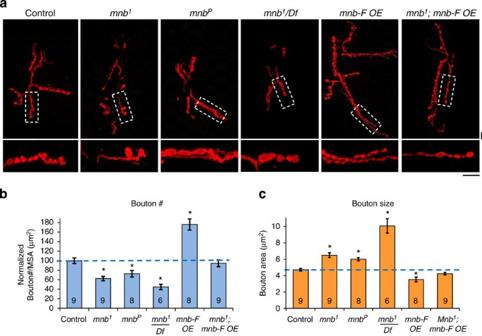Figure 2: Mnb regulates synaptic growth. (a) Muscle 6/7 NMJ at A2 stained by HRP. Lower panels show magnified images of the white boxed region. Scale bar, 10 μm. (b) Number of boutons normalized to muscle surface area (MSA). (c) Average Type Ib bouton area. *P<0.05 compared with control. Sample values are indicated in the bars. All values are mean±s.e.m. Figure 2: Mnb regulates synaptic growth. ( a ) Muscle 6/7 NMJ at A2 stained by HRP. Lower panels show magnified images of the white boxed region. Scale bar, 10 μm. ( b ) Number of boutons normalized to muscle surface area (MSA). ( c ) Average Type Ib bouton area. * P <0.05 compared with control. Sample values are indicated in the bars. All values are mean±s.e.m. Full size image Mnb is required for rapid synaptic vesicle recycling Phosphorylation of synaptic proteins has been proposed as a major mechanism that dynamically regulates the complex protein interactions and enzymatic activities required to maintain stable synaptic transmission [1] , [2] , [3] , [4] , [5] . To determine the importance of Mnb in synaptic function, we performed electrophysiology at the NMJ. We observed that mnb 1 mutants have increased miniature excitatory postsynaptic potential (mEPSP) amplitude but normal evoked EPSP amplitudes ( Fig. 3a–d ), similar to electrophysiological properties observed in other endocytic mutants [33] , [34] , [36] , [40] , [44] . As an increase in mEPSP amplitude could be due to either a postsynaptic change (receptor abundance or activity) or a presynaptic change (such as synaptic vesicle size), we stained the NMJ with an antibody against glutamate receptor IIA (GluRIIA). We observed normal postsynaptic GluRIIA staining in mnb 1 compared with controls, supporting the notion that increases in mEPSP amplitude is due to presynaptic changes ( Supplementary Fig. 2 ). Consistent with this finding, presynaptic overexpression of mnb-F in mnb 1 background ( mnb 1 ; mnb-F OE ) rescued the mEPSP phenotype and that an increase in synaptic vesicle size has been found in a variety of endocytic mutants [33] , [34] , [36] , [40] , [44] . 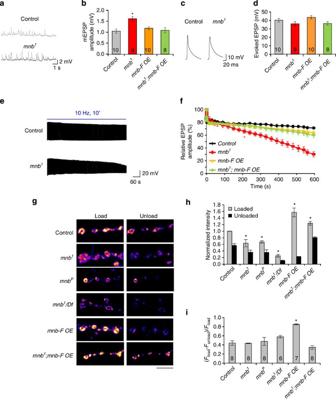Figure 3: Mnb is required for rapid synaptic vesicle recycling. (a) Representative mEPSP. (b) Average mEPSP amplitude. Sample values are indicated in the graph. (c) Representative evoked EPSP and (d) average evoked EPSP. (e) EPSP recordings during 10 Hz stimulation for 10 min. (f) Relative EPSP amplitude plotted over time for the indicated genotypes.n=6 for each genotype. *P<0.05 at the indicated time and beyond compared with control. (g) Images of NMJs after FM1-43 loading and unloading. Scale bar, 10 μm. (h) FM1-43 dye loading and unloading intensity. (i) Quantification of FM1-43 signal removed during unloading normalized to amount of loading. Forhandi,nis indicated in the bar graph ini, *P<0.05 compared with control. All values represent mean±s.e.m. Figure 3: Mnb is required for rapid synaptic vesicle recycling. ( a ) Representative mEPSP. ( b ) Average mEPSP amplitude. Sample values are indicated in the graph. ( c ) Representative evoked EPSP and ( d ) average evoked EPSP. ( e ) EPSP recordings during 10 Hz stimulation for 10 min. ( f ) Relative EPSP amplitude plotted over time for the indicated genotypes. n =6 for each genotype. * P <0.05 at the indicated time and beyond compared with control. ( g ) Images of NMJs after FM1-43 loading and unloading. Scale bar, 10 μm. ( h ) FM1-43 dye loading and unloading intensity. ( i ) Quantification of FM1-43 signal removed during unloading normalized to amount of loading. For h and i , n is indicated in the bar graph in i , * P <0.05 compared with control. All values represent mean±s.e.m. Full size image Interestingly, when we stimulated the nerve at a high frequency (10 Hz) for a prolonged period (10 min), mnb 1 showed significantly faster rundown than controls ( Fig. 3e,f ). This result suggests that Mnb promotes efficient synaptic vesicle recycling during conditions of high activity. Presynaptic overexpression of mnb-F alone did not affect basal synaptic transmission and responses to high-frequency stimulation as compared with the control, but restored maintenance of synaptic transmission when expressed in mnb 1 mutant background ( Fig. 3a–f ). Together, these data indicate neuronal Mnb is required for rapid synaptic vesicle recycling. To directly measure the recycling synaptic vesicle pool, we loaded the synaptic terminals with the lipophilic dye FM1-43 during stimulation, which incorporates into synaptic vesicles during endocytosis and can subsequently be released during exocytosis. The fluorescence intensity corresponds to the net amount of FM1-43 uptake, a function of both exocytosis and endocytosis. Synaptic vesicles of mnb 1 loaded with FM1-43 during 5-min depolarization using high extracellular potassium (60 mM) displayed a significant decrease in FM1-43 loading intensity ( Fig. 3g,h ), indicating a defect in synaptic transmission consistent with the electrophysiology data obtained for prolonged stimulation. mnb P allele showed a similar decrease in loading intensity and mnb 1 /Df showed the most dramatic decrease in FM1-43 loading. To further delineate whether this is due to an endocytic or exocytic defect, we stimulated the loaded boutons again to measure the extent of exocytosis. Figure 3h,i show that mnb mutants have normal exocytosis, as the amount of FM1-43 that unloaded (signal remaining after unloading subtracted from signal from loading) normalized to the amount of loaded was unaltered, thus indicating Mnb reduction causes a specific defect in endocytosis. Interestingly, overexpression of mnb in neurons led to increased FM1-43 loading, while the amount of FM1-43 unloaded was also enhanced ( Fig. 3h,i ). Together with electrophysiology data indicating normal basal synaptic transmission and normal rundown during prolonged high frequency stimulation, the FM1-43 experiments suggest that rates of endocytosis and exocytosis are both enhanced but balanced when Mnb is upregulated. Restoring Mnb level by overexpressing Mnb in mnb 1 compensated for the decrease in FM1-43 loading, consistent with the electrophysiology data. Together, these results confirm that Mnb facilitates rapid synaptic vesicle endocytosis. Synj is a substrate of Mnb Dyrk1A/Mnb has been shown to phosphorylate a number of endocytic proteins including Synj and dynamin in vitro [25] , [26] , but there is a lack of in vivo evidence and the physiological consequence of Dyrk1A/Mnb-mediated phosphorylation are not well understood. We therefore tested the possibility that Synj is a potential substrate of Mnb. We first determined whether Mnb can biochemically interact with Synj by performing immunoprecipitation. Mnb-F was detected in the pull-down with Synj and vice versa ( Fig. 4a and Supplementary Fig. 3a ), indicating that Mnb can bind to Synj. We also observed partial colocalization between Mnb and haemagglutinin (HA)-tagged Synj within the fly NMJ ( Fig. 4b ). 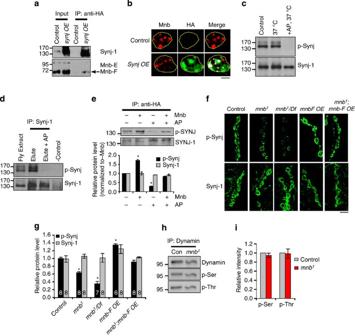Figure 4: Mnb binds to and phosphorylates Synj bothin vitroandin vivo. (a) Immunoprecipitation (IP) experiment using flies overexpressing Synj tagged with HA reveals that Synj interacts with Mnb-F. Control: wild-type flies without Synj-HA overexpression. (b) Image of an individual bouton stained with Mnb and HA antibodies. Mnb colocalizes with Synj-HA in the presynaptic terminal of flies overexpressing HA-tagged Synj (highlighted by white pixels). Scale bar, 2 μm. (c) AP treatment shows that the p-Synj antibody has significantly greater affinity for phospho-Synj. (d) IP done using Synj-1 antibody followed by AP treatment reveals that Synj-1 can also detect both phosphorylated and non-phosphorylated Synj. ‘–control’ indicates parallel IP performed using IgG as negative control instead of Synj antibody. (e) Incubation of immunoprecipitated Synj in the presence and absence of AP and Mnb. Pre-treatment of Mnb enhanced Synj phosphorylation as revealed by p-Synj antibody. Lower graph shows quantification of relative p-Synj and Synj-1 signals in the indicated treatment conditions.n=3, *P<0.05 as compared with control. (f) Staining of Synj in the third instar NMJ done using p-Synj and Synj-1 antibodies for the indicated genotypes.mnboverexpression increased p-Synj staining in the synapse while Mnb reduction in mutants decreased the level of p-Synj. Scale bar=10 μm. (g) Quantification of relative staining intensity for p-Synj and Synj-1 signals. n is indicated in the bar graph, * indicatesP<0.05 as compared to control. (h) IP done using dynamin antibody, and the levels of phospho-serine (p-Ser) and phospho-threonine (p-Thr) were determined using phospho-specific antibodies as indicated. (i) Quantification of relative levels of p-Ser and p-Thr after normalizing to the amount of dynamin in the IP.n=3. All values represent mean±s.e.m. Figure 4: Mnb binds to and phosphorylates Synj both in vitro and in vivo . ( a ) Immunoprecipitation (IP) experiment using flies overexpressing Synj tagged with HA reveals that Synj interacts with Mnb-F. Control: wild-type flies without Synj-HA overexpression. ( b ) Image of an individual bouton stained with Mnb and HA antibodies. Mnb colocalizes with Synj-HA in the presynaptic terminal of flies overexpressing HA-tagged Synj (highlighted by white pixels). Scale bar, 2 μm. ( c ) AP treatment shows that the p-Synj antibody has significantly greater affinity for phospho-Synj. ( d ) IP done using Synj-1 antibody followed by AP treatment reveals that Synj-1 can also detect both phosphorylated and non-phosphorylated Synj. ‘–control’ indicates parallel IP performed using IgG as negative control instead of Synj antibody. ( e ) Incubation of immunoprecipitated Synj in the presence and absence of AP and Mnb. Pre-treatment of Mnb enhanced Synj phosphorylation as revealed by p-Synj antibody. Lower graph shows quantification of relative p-Synj and Synj-1 signals in the indicated treatment conditions. n =3, * P <0.05 as compared with control. ( f ) Staining of Synj in the third instar NMJ done using p-Synj and Synj-1 antibodies for the indicated genotypes. mnb overexpression increased p-Synj staining in the synapse while Mnb reduction in mutants decreased the level of p-Synj. Scale bar=10 μm. ( g ) Quantification of relative staining intensity for p-Synj and Synj-1 signals. n is indicated in the bar graph, * indicates P <0.05 as compared to control. ( h ) IP done using dynamin antibody, and the levels of phospho-serine (p-Ser) and phospho-threonine (p-Thr) were determined using phospho-specific antibodies as indicated. ( i ) Quantification of relative levels of p-Ser and p-Thr after normalizing to the amount of dynamin in the IP. n =3. All values represent mean±s.e.m. Full size image To further examine the extent to which Mnb influences the phosphorylation state of Synj phosphorylation, we obtained an antibody against the PRD of Drosophila Synj [30] . On alkaline phosphatase (AP) treatment, we found that this antibody has a greater preference for the phosphorylated form of Synj, as no signal was detected following AP treatment using this antibody ( Fig. 4c ; p-Synj). Note that the lack of signal is not due to protein degradation, as Synj is still detected using another antibody generated against part of the SAC-1 domain of Synj ( Fig. 4c ; Synj-1). To further ensure that Synj-1 antibody is specific for Synj, we immunoprecipitated Synj using Synj-1 and detected the eluate with both the p-Synj and Synj-1 antibodies. Figure 4d shows that the Synj-1 antibody is specific for Synj, and can detect both the phosphorylated and non-phosphorylated form of Synj. We took advantage of these independent Synj antibodies to test whether Mnb can directly phosphorylate Synj. We pre-treated purified Synj expressed in bacteria with AP, which removed most of the existing phosphorylation, and then incubated Synj with purified His-Mnb protein. Addition of purified Mnb significantly increased p-Synj signal while total Synj level remain unchanged ( Supplementary Fig. 3b ), indicating that Mnb can indeed directly phosphorylate Synj. Interestingly, we noticed that Synj expressed in bacteria has Mnb phosphorylation site(s) already saturated, as addition of Mnb without AP treatment failed to increase Synj phosphorylation detected by p-Synj antibody ( Supplementary Fig. 3c ). As phosphorylation of Synj in Escherichia Coli is unexpected, we performed mass spectrometry to determine the presence of phosphorylation sites in the PRD of purified Synj. Supplementary Fig. 3d shows that Synj purified from bacteria has 11 sites with >75% probability of being phosphorylated. This may explain why the p-Synj antibody originally generated using the PRD of Synj purified from bacteria as immunogen preferentially recognizes the phosphorylated form of Synj. Addition of purified Mnb to Synj immunocipitated from fly extracts also significantly increased p-Synj signal with or without prior AP treatment ( Fig. 4e ), confirming that Synj is a substrate of Mnb and further implying dynamic regulation of Synj phosphorylation by Mnb. Having demonstrated that Mnb can bind to and phosphorylate Synj, we next asked whether synaptic Synj phosphorylation levels depend on Mnb. We found that mnb 1 displayed a significant decrease in the level of phospho-Synj, while the total level of Synj as detected by Synj-1 remains unchanged ( Fig. 4f, g ). mnb 1 /Df showed a further decrease in Synj phosphorylation, whereas mnb overexpression in neurons caused a significant increase in phospho-Synj level locally within the synaptic terminals. Upregulating Mnb in mnb 1 background restored Synj phosphorylation to normal levels ( Fig. 4f, g ), confirming that Mnb regulates Synj phosphorylation levels in vivo . Similar results were obtained via western blottng analyses using antibodies against p-Synj and Synj-1 ( Supplementary Fig. 3e,f ). We also examined the overall serine and threonine phosphorylation status of immunoprecipitated Synj using phospho-serine- and phospho-threonine-specific antibodies. We observed a reduction in the levels of both phospho-serine and phospho-threonine in mnb 1 flies ( Supplementary Fig. 3g ) Taken together, our data suggest that Mnb is a synaptic kinase that regulates Synj phosphorylation. We next examined the possibility that Mnb phosphorylates other endocytic proteins to regulate synaptic vesicle recycling. To this end, we purified or enriched for phosphorylated proteins from fly heads with phosphoprotein purification columns, which offers the advantage of simultaneous isolation of proteins phosphorylated on the serine, threonine and tyrosine residues [45] , as well as systematic detection of the level of different phosphorylated and non-phosphorylated proteins using western blotting analyses. We find mnb mutation did not reduce the phosphorylation of dynamin, Endo, or Dap160 ( Supplementary Fig. 3h ). As dynamin was previously shown to be a substrate of Dyrk1A/Mnb in vitro [26] , we further validated these results by immunoprecipitating dynamin from control and mnb 1 flies, and determined the extent of dynamin phosphorylation using phospho-serine- or phospho-threonine-specific antibodies. We found mnb 1 flies displayed normal levels of dynamin phosphorylated on the serine and threonine residues ( Fig. 4h, i ). Thus, Mnb is not likely to influence endocytosis through altered phosphorylation of dynamin, Endo, or Dap160, and Synj is a specific endocytic substrate in vivo . Mnb phosphorylation of Synj alters protein interactions The PRD at the carboxy terminus of Synj is capable of binding to multiple endocytic proteins with SH3 domains such as Endo and Dap160 to couple synaptic vesicle fission and uncoating [28] , [29] , [30] , [32] , [33] , [34] . Furthermore, it was shown that phosphorylation of Synj within the PRD by kinases such as Cdk-5 and Ephrin receptor negatively regulates its interaction with Endo [37] , [38] , but the effect of Mnb phosphorylation on endocytic protein interactions is unclear. Pull-down studies using Synj-HA expressed in bacteria revealed that Mnb incubation (following pre-treatment with AP) not only increased the level of Synj phosphorylation, but also reduced Synj interactions with Endo while increasing Dap160 interactions ( Supplementary Fig. 4a,b ). This result suggests that Mnb-dependent phosphorylation of Synj shifts its interaction preference to Dap160. To further establish the importance of Mnb-dependent phosphorylation in vivo , we examined Synj interaction using immunoprecipitation studies. We observed that mnb 1 mutants exhibited increased Synj–Endo interaction but reduced Dap160 binding as compared with the control ( Fig. 5a,b ), indicating that Mnb alters the endocytic scaffold complex and may act to regulate recruitment of Synj during clathrin-mediated endocytosis. To confirm that this decrease in Synj-Dap160 is not due to altered Dap160 level, which is an important scaffolding protein required for proper localization of endocytic proteins, we also immunostained the NMJs with Dap160 antibody in control, mnb 1 and mnb 1 /Df lines ( Supplementary Fig. 4c,d ). Note that no change was observed, and the levels of Endo and Syt are also normal. 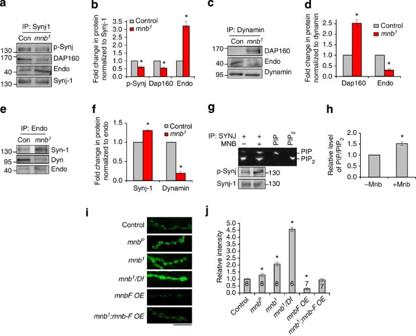Figure 5: Mnb regulates endocytic protein interactions and enhances Synj 5′-phosphoinositol phosphatase activity. (a) Immunoprecipitation (IP) performed using Synj-1 antibody, (c) IP performed using dynamin antibody and (e) IP done using Endo antibody followed by western blottings of the IP eluates done using the indicated antibodies. (b,d,f) Quantification of protein levels detected in themnb1IP eluate as compared with control.n=3 independent experiment. (g) TLC showing conversion of BODIPY-PIP2 to BODIPY-PIP by Synj-HA immunoprecipitated from fly extracts with and without addition of purified Mnb protein. Lower panels show levels of phospho-Synj and total Synj as detected by p-Synj and Synj-1 antibodies, respectively. (h) Quantification of relative PIP to PIP2level.n=4 independent experiments. (i) PIP2levels in the NMJ as measured by PLCδ1-PH-GFP for the indicated genotypes. Scale bar, 10 μm. (j) Quantification of PIP2levels in the synapse. Lower Synj activity results in reduced conversion of PIP2to PIP, and will hence have higher PIP2levels detected by PLCδ1-PH-GFP in the synapse. Sample numbers are indicated in the bar graph. *P<0.05 forb,d,f,handjas compared with the respective control. All values are mean±s.e.m.. Figure 5: Mnb regulates endocytic protein interactions and enhances Synj 5′-phosphoinositol phosphatase activity. ( a ) Immunoprecipitation (IP) performed using Synj-1 antibody, ( c ) IP performed using dynamin antibody and ( e ) IP done using Endo antibody followed by western blottings of the IP eluates done using the indicated antibodies. ( b , d , f ) Quantification of protein levels detected in the mnb 1 IP eluate as compared with control. n =3 independent experiment. ( g ) TLC showing conversion of BODIPY-PIP2 to BODIPY-PIP by Synj-HA immunoprecipitated from fly extracts with and without addition of purified Mnb protein. Lower panels show levels of phospho-Synj and total Synj as detected by p-Synj and Synj-1 antibodies, respectively. ( h ) Quantification of relative PIP to PIP 2 level. n =4 independent experiments. ( i ) PIP 2 levels in the NMJ as measured by PLCδ1-PH-GFP for the indicated genotypes. Scale bar, 10 μm. ( j ) Quantification of PIP 2 levels in the synapse. Lower Synj activity results in reduced conversion of PIP 2 to PIP, and will hence have higher PIP 2 levels detected by PLCδ1-PH-GFP in the synapse. Sample numbers are indicated in the bar graph. * P <0.05 for b , d , f , h and j as compared with the respective control. All values are mean±s.e.m.. Full size image As the PRD of either Synj or dynamin binds to a single SH3 domain of Endo [28] , [30] , [40] , [46] , we further examined the possibility that altered Synj phosphorylation may influence the dynamic equilibrium between dynamin and Endo in vivo . Interestingly, mnb 1 mutants showed reduced interaction between Endo and dynamin ( Fig. 5c,d ). This result was further confirmed by immunoprecipitation performed using Endo antibody ( Fig. 5e,f ), which confirmed reduced interaction between Endo and dynamin, but enhanced Endo–Synj-1 interaction in mnb 1 as compared with control. Collectively, these data demonstrate that Mnb-mediated Synj phosphorylation modulates the balance between key endocytic protein interactions, perhaps to ensure robust and rapid endocytosis during periods of high activity. Synj enzymatic activity is enhanced by Mnb phosphorylation Synj is a phosphoinositol phosphatase capable of regulating PI(4,5)P 2 levels, which modulates endocytosis and synaptic growth [30] , [31] , [36] , [37] , [47] , [48] , [49] , [50] . Thus, we tested the hypothesis that phosphorylation of Synj by Mnb alters Synj phosphoinositol phosphatase activity. We found that the addition of purified Mnb, which has been shown to directly phosphorylate Synj, increased the 5′-phosphatase activity of immunoprecipitated Synj in vitro as assayed by increased conversion of BODIPY-labelled PI(4,5)P 2 to BODIPY-PI(4)P using thin layer chromatography ( Fig. 5g,h ). This finding indicates that Mnb-mediated phosphorylation of Synj directly enhances Synj activity. To test whether Mnb phosphorylation indeed influences Synj activity in vivo amid complex kinase and phosphatase signalling, we examined Synj activity in mnb mutants using two complementary approaches. First, phosphoinositol 5′-phosphatase activity was determined from control and mnb mutant extracts using TLC. mnb 1 and mnb 1 /Df flies exhibited lower levels of converted PI(4,5)P 2 ( Supplementary Fig. 4e,f ), confirming that the overall Synj activity is reduced in flies with lower Mnb expression levels. This decrease in Synj activity parallels reduced Synj phosphorylation levels ( Supplementary Fig. 3e,f ), consistent with enhancement of Synj activity by Mnb. Second, to determine whether Mnb regulates Synj activity locally at the synapse, we used the enhanced green fluorescent protein (GFP) fusion protein containing the phospholipase Cδ1 pleckstrin homology domain (PLCδ1-PH-GFP) [50] . PLCδ1-PH-GFP has been shown to specifically bind to PI(4,5)P 2 , and the fluorescence intensity in the synapse directly reflects the level of PI(4,5)P 2 . NMJs were labelled with HRP to outline synaptic boutons and the intensity of the PLCδ1-PH-GFP signal was examined for different mnb mutants. Consistent with our hypothesis, we find higher PLCδ1-PH-GFP signal in mnb 1 and mnb 1 /Df NMJs, implying lower Synj activity locally within the NMJ ( Fig. 5i,j ). Overexpression of Mnb-F decreased PLCδ1-PH-GFP signal in the synaptic boutons, suggesting Mnb upregulation leads to elevated Synj activity. Upregulating Mnb-F in mnb 1 restored PLCδ1-PH-GFP signal to normal, confirming that Mnb is responsible for changes in PI(4,5)P 2 levels. To further establish that Mnb alters PI(4,5)P2 levels by acting through Synj in vivo , we reduced the level of Synj in flies overexpressing mnb-F ( synj 1 /mnbC-F OE ). Although mnb overexpression significantly reduced the PLCδ1-PH-GFP signal, decreasing the level of Synj in a mnb overexpression background was sufficient to restore PLCδ1-PH-GFP levels ( Supplementary Fig. 4g,h ). Reduction of Synj alone ( synj 1 /+) resulted in a slight elevation in PLCδ1-PH-GFP signal, consistent with a previous report [51] . Taken together, our results suggest that Mnb phosphorylation of Synj enhances its phosphoinositol phosphatase activity and is required for normal PI(4,5)P 2 in the synapse. Mnb phosphorylates and enhances Synj during synaptic activity Having demonstrated that Mnb can phosphorylate and potentiate Synj activity, we next asked whether Mnb acts during synaptic stimulation to correspondingly facilitate endocytosis through Synj. To this end, we first determined Mnb localization within the synapse at rest and after synaptic stimulation induced by high KCl ( Fig. 6a ). Compared with unstimulated synapses, colocalization between Mnb and Endo increased during synaptic activity, while colocalization with BRP was unchanged ( Fig. 6b ). This result suggests that synaptic activity further mobilizes Mnb to the periactive zone. Next, we examined whether Mnb redistribution influences Mnb-mediated phosphorylation of Synj by immunocytochemistry using antibodies against p-Synj and Synj-1 ( Fig. 6c ). Although Synj-1 levels in control were the same at rest and following synaptic activity, synaptic activity increased the level of p-Synj in the synapse ( Fig. 6c ). This result demonstrates that Synj phosphorylation levels are enhanced by synaptic activity. To determine whether Mnb is responsible for this activity-dependent increase in Synj phosphorylation, we compared the percent increase in p-Synj levels after stimulation between control, mnb 1 and mnb 1 /Df. We observed a smaller enhancement of p-Synj in mnb 1 and mnb 1 /Df compared with the control ( Fig. 6d ), confirming that Mnb is required for full Synj phosphorylation during synaptic activity. 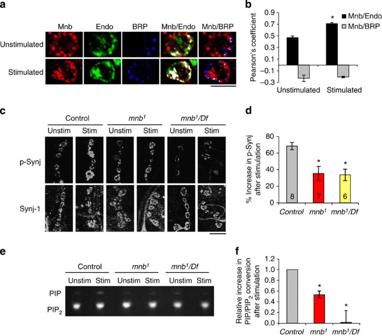Figure 6: Synaptic activity promotes Mnb-dependent Synj phosphorylation and activity enhancement. (a) Images of synaptic bouton triple-labelled for Endo, Mnb and BRP at rest and after stimulation with high K+for 30 s. Colocalization is highlighted by white pixels. Scale bar, 2 μm. (b) Pearson’s correlation coefficient values showing colocalization between Mnb/Endo but not Mnb/BRP. Stimulation enhanced colocalization between Mnb and Endo.n=5 independent experiment per condition. *P<0.05 compared with unstimulated bouton. (c) Images of NMJs stained with p-Synj or Synj-1 antibodies at rest (unstim) and stimulated (stim) with high K+. Scale bar, 10 μm. (d) Quantification of the increase in p-Synj level after stimulation, normalized to total Synj level. Compared with control,mnb1andmnb1/Dfshow a lower level of increase in phospho-Synj after stimulation.nis indicated in the bars. *P<0.05 compared with control. (e) TLC showing conversion of BODIPY-PIP2 to BODIPY-PIP by larval extract with and without stimulation with high K+. (f) Quantification of the increase in PIP2conversion after stimulation.n=3 independent experiments. *P<0.05 compared with control. All values represent mean±s.e.m. Figure 6: Synaptic activity promotes Mnb-dependent Synj phosphorylation and activity enhancement. ( a ) Images of synaptic bouton triple-labelled for Endo, Mnb and BRP at rest and after stimulation with high K + for 30 s. Colocalization is highlighted by white pixels. Scale bar, 2 μm. ( b ) Pearson’s correlation coefficient values showing colocalization between Mnb/Endo but not Mnb/BRP. Stimulation enhanced colocalization between Mnb and Endo. n =5 independent experiment per condition. * P <0.05 compared with unstimulated bouton. ( c ) Images of NMJs stained with p-Synj or Synj-1 antibodies at rest (unstim) and stimulated (stim) with high K + . Scale bar, 10 μm. ( d ) Quantification of the increase in p-Synj level after stimulation, normalized to total Synj level. Compared with control, mnb 1 and mnb 1 /Df show a lower level of increase in phospho-Synj after stimulation. n is indicated in the bars. * P <0.05 compared with control. ( e ) TLC showing conversion of BODIPY-PIP2 to BODIPY-PIP by larval extract with and without stimulation with high K + . ( f ) Quantification of the increase in PIP 2 conversion after stimulation. n =3 independent experiments. * P <0.05 compared with control. All values represent mean±s.e.m. Full size image We next tested whether Mnb-mediated phosphorylation of Synj influences Synj 5′-phosphoinositol phosphatase activity during synaptic stimulation. Consistent with our finding that phosphorylation enhances Synj activity, larval extracts isolated from control before and after stimulation showed a higher level of PI(4,5)P 2 conversion after stimulation ( Fig. 6e ), indicating synaptic stimulation augments Synj activity. However, mnb 1 and mnb 1 /Df showed little or no enhancement in Synj activity after stimulation, indicating that Mnb critically modulates Synj activity during synaptic stimulation ( Fig. 6f ). Interestingly, although mnb 1 /Df showed almost no Synj activity enhancement as compared with mnb 1 ( Fig. 6f ), the level of change in p-Synj was comparable between the two genotypes ( Fig. 6d ). This implies that Synj is likely to be phosphorylated at multiple sites, but the p-Synj antibody may not be able to distinguish between all the sites. Altogether, our results suggest that Mnb is required for activity-dependent phosphorylation and enhancement of Synj. If Mnb regulates Synj function and in turn facilitates synaptic vesicle endocytosis in response to synaptic activity, then acute inhibition of Mnb may be sufficient to disrupt synaptic vesicle recycling. To test this hypothesis, we pre-treated the larval NMJ with proINDY, a selective and cell-permeable inhibitor of Dyrk1A that had been shown to effectively inhibit Dyrk1A activity in cultured cells at 30 μM [52] . We found incubation of the dissected larval NMJ with proINDY for 30 min before and during stimulation (50 μM proINDY) effectively inhibited FM1-43 loading ( Supplementary Fig. 5a ), suggesting that acute inhibition of Mnb function can disrupt synaptic vesicle recycling. This result is further confirmed by electrophysiological recordings, in which ProINDY-treated samples showed a faster EPSP rundown compared with control NMJ treated with vehicle only (percentage of starting EPSP amplitude 5 min post stimulation: 80.20±3.46% for vehicle control versus 44.47±4.57% for drug treated; P <0.01; n =7). Acute application of ProINDY decreased mEPSP amplitudes in control larvae (1.44±0.21 mV for vehicle control versus 0.91±0.07 mV for drug treated; P <0.04; n =11), suggesting that the increase in mEPSP observed in mnb 1 is a result of chronic developmental perturbations to synaptic vesicle endocytosis. Inhibiting Mnb also reduced the level of phosphorylated Synj in a dose-dependent manner without altering the total level of Synj-1 ( Supplementary Fig. 5b,c ). Together, these results are consistent with Mnb function being required acutely to promote efficient synaptic vesicle recycling. Synj upregulation compensates for loss of Mnb activity Based on findings that mnb 1 displayed reduced Synj activity, we hypothesized that increasing Synj expression may elevate Synj activity and therefore rescue mnb 1 phenotypes. We first confirmed the levels of phospho-Synj and total Synj level in flies overexpressing synj alone ( synj OE) or Synj in mnb 1 background ( mnb 1 ; synj OE; Supplementary Fig. 6a,b ). Overexpression of Synj dramatically increased the level of phospho-Synj, while overexpression of Synj in mnb 1 background reduced the level of phospho-Synj compared with synj OE in an otherwise wild-type background. However, the level of phosphorylated Synj is still elevated, likely to be due to residual Mnb function in the hypomorphic mnb 1 allele. In addition, we measured the relative PI(4,5)P 2 levels within the NMJ using PLCδ1-PH-GFP as an in vivo readout of Synj enzymatic activity ( Fig. 7a,b ). Consistent with the level of phosphorylated Synj, we found that mnb 1 ; synj OE significantly rescued the mnb 1 phenotype in terms of PI(4,5)P 2 intensity. Immunostaining of the NMJ with HRP revealed that Synj upregulation in mnb 1 restored the bouton size, but not the number of boutons ( Supplementary Fig. 6c–e ), indicating that Mnb-dependent modulation of Synj activity regulates size, and not the number of boutons. This result is further supported by experiments in which overexpression of PLCδ1-PH-GFP, which was also used to locally deplete PI(4,5)P 2 (refs 50 , 53 ), effectively restored bouton size but did not alter the number of boutons ( Supplementary Fig. 6f,g ). 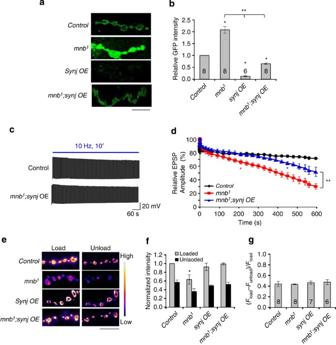Figure 7: Upregulation of Synj rescues defective endocytosis inmnb1. (a) Representative images of PIP2levels in the NMJ as measured by PLCδ1-PH-EGFP for the indicated genotypes. Scale bar, 10 μm. (b) Quantification of PIP2levels. Synj overexpression inmnb1has lower PI(4,5)P2level thanmnb1in the synapse, suggesting a rescue of Synj activity. Sample numbers are indicated in the bars. *P<0.05 compared with control and **P<0.05 as indicated. (c) Representative EPSP traces during 10 Hz stimulation for the indicated genotypes. (d) Relative EPSP amplitude plotted over time for the indicated genotypes.n=6 and *P<0.05 from the indicated time point and beyond as compared with control. **P<0.05 as compared withmnb1. (e) Images of NMJ after FM1-43 loading and unloading. Scale bar, 10 μm. (f) Relative FM1-43 loading and unloading intensity normalized to control. *P<0.05 compared with control. (g) Quantification of FM1-43 signal removed during unloading normalized to amount of loading. Forfandg,nis indicated in the bar graph in (g). All values represent mean±s.e.m. Figure 7: Upregulation of Synj rescues defective endocytosis in mnb 1 . ( a ) Representative images of PIP 2 levels in the NMJ as measured by PLCδ1-PH-EGFP for the indicated genotypes. Scale bar, 10 μm. ( b ) Quantification of PIP 2 levels. Synj overexpression in mnb 1 has lower PI(4,5)P 2 level than mnb 1 in the synapse, suggesting a rescue of Synj activity. Sample numbers are indicated in the bars. * P <0.05 compared with control and ** P <0.05 as indicated. ( c ) Representative EPSP traces during 10 Hz stimulation for the indicated genotypes. ( d ) Relative EPSP amplitude plotted over time for the indicated genotypes. n =6 and * P <0.05 from the indicated time point and beyond as compared with control. ** P <0.05 as compared with mnb 1 . ( e ) Images of NMJ after FM1-43 loading and unloading. Scale bar, 10 μm. ( f ) Relative FM1-43 loading and unloading intensity normalized to control. * P <0.05 compared with control. ( g ) Quantification of FM1-43 signal removed during unloading normalized to amount of loading. For f and g , n is indicated in the bar graph in ( g ). All values represent mean±s.e.m. Full size image Our previous results have shown that overexpression of synj alone does not influence synaptic vesicle recycling [54] , we thus next tested the ability of synj overexpression to restore the endocytic defect seen in mnb 1 mutants. We find that synj overexpression in mnb 1 background significantly rescued the faster rundown phenotype seen in mnb 1 during stimulation ( Fig. 7c,d ). However, after prolonged stimulation at 10 Hz (after 450 s of stimulation), we noticed that NMJs with synj overexpression in mnb 1 background also began to display a slightly faster rundown than the control. This is likely due to inefficient phosphorylation and enhancement of Synj activity during synaptic stimulation in mnb 1 background over time, despite the increase in Synj protein level. FM1-43 labelling experiments further confirmed that synj overexpression rescued altered endocytosis in mnb 1 mutant ( Fig. 7e–g ). We also assessed the ability of synj overexpression to rescue defective locomotor response in mnb 1 (ref. 14 ). Consistent with findings that synj overexpression effectively restored Synj phosphorylation and activity, it also restored locomotor activity to normal ( Supplementary Fig. 6h ). Furthermore, presynaptic synj overexpression restored mEPSP amplitudes near control levels (1.04±0.10 mV for control; 1.62±0.11 mV for mnb 1 ; 1.26±0.09 mV for mnb 1 ; synj OE . P =0.11 for control versus mnb 1 ;synj OE ; P =0.03 for mnb 1 versus mnb 1 ;synj OE ; n =9 per genotype). Interestingly, although synj overexpression significantly rescued the synaptic phenotypes seen in mnb 1 , it did not restore the decrease in brain size seen in mnb 1 ( Supplementary Fig. 6i ), suggesting this function of Mnb is independent of Synj phosphorylation. These results demonstrate that Mnb has multiple roles in the nervous system and that it probably acts locally within the synapse to phosphorylate Synj and couple synaptic vesicle endocytosis to neural activity. We demonstrate that Mnb is a novel synaptic kinase essential for normal synaptic morphology and synaptic vesicle endocytosis, and that function is largely subserved through phosphorylation of the synaptic endocytosis protein Synj. Furthermore, our data revealed a new role for Dyrk1A/Mnb in the synapse, both in regulating Synj 5′-phosphoinositol phosphatase activity and in coordinating interactions between Synj and other endocytic proteins. Our observations of increased colocalization of Mnb with endocytic markers and elevated levels of phosphorylated Synj during synaptic activity further support the notion that Mnb acts during neuronal stimulation to enhance Synj function to sustain neurotransmission during periods of high demand. Interestingly, Cdk5 and ephrin receptor kinase have been shown to inhibit Synj through phosphorylation [37] , [38] , while we find that the effect of Mnb phosphorylation on Synj activity is stimulatory. One attractive model, therefore, is that these kinases along with phosphatases bidirectionally control Synj activity and, in turn, endocytic efficiency. Current models for synaptic vesicle endocytosis suggest that intricately coordinated interactions between distinct endocytic proteins are essential for normal synaptic vesicle recycling [55] . Although the precise timing of biochemical interactions during different steps is not well understood, it was suggested that Dap160/intersectin is an important scaffolding protein that maintains dynamin, Synj and Endo at the periactive zone [29] , [33] , [34] , [56] , that Endo–dynamin interaction facilitates localization of dynamin at the neck of the clathrin-coated pits before fission during early-step endocytosis [57] , and that recruitment of Synj by Endo promotes uncoating of clathrin during late endocytosis [30] , [32] , [36] , [58] . Our data demonstrate that mnb mutants did not affect the overall levels of Dap160, Synj and Endo at the NMJ, but shifted the binding preference of Synj to enhance interactions with Endo with concomitant reductions in Dap160–Synj and Endo–dynamin interactions. Thus, phosphorylation of Synj by Mnb probably coordinates endocytic protein interactions to facilitate efficient endocytosis during conditions of high activity. In addition to regulating endocytosis, we found Mnb also influences synaptic growth and morphology. Furthermore, we demonstrate that either reducing or increasing Mnb levels resulted in abnormal synaptic morphology, further highlighting the importance of Mnb dosage in controlling synaptic growth. The increase in synaptic bouton size seen in mnb mutants may be due to its inability to retrieve membrane following exocytosis and/or through altered Synj activity, which governs PI(4,5)P 2 availability in the NMJ. PI(4,5)P 2 has been shown to restrict synaptic growth through activation of presynaptic Wiscott–Aldrich syndrome protein/WASP, which is thought to stimulate actin branching to promote synaptic bouton growth while restricting synapse extension at the NMJ [50] , [59] , [60] , [61] , [62] . In support of the hypothesis that Mnb partially affects synaptic growth through Synj and subsequent PI(4,5)P2 levels, overexpression of Synj in mnb 1 background restored bouton size and that expression of PLCδ1-PH-GFP, which had previously been shown to deplete PI(4,5)P 2 , rescued the change in bouton size in mnb 1 . As reducing Synj phosphorylation and activity in mnb 1 is not physiologically equivalent to an actual loss of Synj protein, the synaptic morphology of mnb 1 was different from synj -null mutants (reported to show either hyperbudding or no change in synaptic morphology) [30] , [63] . Note that although synj overexpression in mnb 1 did rescue synaptic bouton size, it did not restore the number of synaptic boutons to normal levels, implying that Mnb also affects other pathways independently from Synj to influence synaptic morphology. Similar to many of the in vivo substrates identified to be phosphorylated by Dyrk1A, fly Synj does not contain the consensus sequence for Dyrk1A/Mnb phosphorylation, and the PRD does not share sequence similarities with its mammalian orthologue. However, similar to mammalian Synj PRD, fly Synj does contain multiple (S/T)P sites in the PRD that may be phosphorylated by Mnb, which is a proline-directed kinase. Our data reveal that Mnb reduction decreased the levels of Synj phosphorylated both on the serine and threonine residues, indicating that Synj is phosphorylated on multiple sites, consistent with a previous report in vitro [25] . The activity-dependent phosphorylation and enhancement of Synj function by Mnb may provide a mechanism to tune the speed of synaptic vesicle recycling and to adapt to periods of high synaptic activity. It will be particularly interesting to determine in the future factors regulating Mnb in the synapse, identify differential phosphorylation sites regulating Synj function and to elucidate the dynamic biochemical interactions that optimize the speed of vesicle recycling over a range of synaptic activity. Interestingly, disturbances in Synj and Dyrk1A have been linked to a number of neurological diseases. Mutations in Dyrk1A/Mnb and Synj have recently been reported in autism [8] , [9] and Parkinson’s disease [64] , respectively. Furthermore, both Synj and Dyrk1A are upregulated in Down syndrome [7] , [65] , [66] . synj overexpression in Down syndrome is thought to contribute to endosomal defects and cognitive deficits [47] , [67] , and Dyrk1a/mnb is a strong candidate gene for learning disabilities [10] , [11] , [19] . Our findings that Dyrk1A/Mnb interacts and enhances Synj function further raises the interesting possibility that co-upregulation of both Dyrk1A/Mnb and Synj may functionally interact and perhaps contribute to some of the Down syndrome phenotypes. An understanding of Dyrk1A/Mnb-dependent regulation of Synj in modulating synaptic growth and neurotransmission thus may not only provide valuable information on fundamental mechanisms controlling endocytosis, but also shed light on cellular mechanisms leading to dysfunctional synapses in these neurological disorders. Fly stocks and antibody generation Flies were cultured at 25 °C on standard cornmeal, yeast, sugar and agar medium. The following fly lines were used: mnb 1 (ref. 14 ), mnb f0137 (abbreviated mnb P in this manuscript; Exelixis Collection, Harvard Medical School), Df (6217; Bloomington Stock Center, Indiana University) and UAS-PLCδ1-PH-GFP [51] . The synj and mnb-F transgene constructs were generated by subcloning the coding regions of synj or mnb-F into the pINDY6 vector, which contains the HA tag, and transgenic flies were generated by standard transformation method. To drive neuronal expression, n-synaptobrevin-Gal4 (n Syb-Gal4 ) [68] was used (gift from Julie Simpson). Affinity-purified rabbit polyclonal antibody for Mnb was generated against Mnb-F amino acids 21–151, a region that is conserved between all Mnb isoforms, and for Synj was generated against amino acids 361–535 (PrimmBiotech, Inc.). All other stocks and standard balancers were obtained from Bloomington Stock Center (Bloomington, IN). Immunochemistry Third-instar larvae were dissected and fixed in 4% paraformaldehyde (except Bouin’s fixative was used for GluRIIA staining). Fixed samples were washed with 0.1% triton X-100 in PBS then blocked with 5% normal goat serum in 0.1% triton X-100 in PBS. Primary antibodies used to label dissected larvae were diluted in blocking solution and used as follows: rabbit anti-p-Synj, 1:2,000 (ref. 30 ); guinea-pig anti-Endo(GP69), 1:200 (ref. 40 ), guinea-pig anti-Dap160, 1:1,000 (ref. 33 ); rabbit anti-synaptotagmin, 1:1,000 (ref. 69 ), rabbit anti-Mnb, 1:400; rabbit anti-Synj-1, 1:200; mouse anti-dynamin, 1:200 (BD Transduction Laboratories); Cy3-conjugated anti-HRP, 1:100 (Jackson ImmunoResearch); mouse anti-BRP (NC82), 1:10; mouse anti-GluRIIA, 1:50; and mouse anti-Dlg (4F3), 1:500 (Developmental Studies Hybridoma Bank). Secondary antibodies used were Alexa-488, 555 or 405 conjugated, 1:250 (Invitrogen). Image quantification Images of synaptic terminals from NMJ 6/7 in A2 were captured using a Zeiss LSM5 confocal microscope using a × 63 1.6 numerical aperture oil-immersion objective. Bouton number was determined by counting the number of HRP-labelled terminals and then normalizing it to the surface area of muscle 6/7 taken with a × 10 objective. Average bouton size was determined by manually circling individual bouton using Image J. Staining intensities were calculated by normalizing the fluorescence intensity to outlined bouton area using AxioVs40 4.8.2.0 or Image J. When comparing intensity across genotypes, the exposure time was kept constant for all genotypes per experiment. All values were normalized to control done within the same experimental set. Electrophysiology Electrophysiology was performed using an Olympus BX51W1 fixed stage microscope equipped with a × 40 0.8 numerical aperture water-dipping objective. Third-instar larvae were dissected and then bathed in a modified HL-3 saline (in mM): NaCl 70, KCl 5, MgCl 2 10, NaHCO 3 10, sucrose 115, trehalose 5, HEPES 5 (pH 7.2) and 0.5 or 2 mM CaCl 2 added as indicated. Current-clamp recordings were performed on muscles 6 or 7 in abdominal segments A2, A3 or A4, and severed ventral nerves were stimulated with suction electrodes at 3-ms stimulus duration. A recording electrode (15–30 MΩ resistance) filled with 3 M KCl was used and data was only analysed from muscles with a resting potential more hyperpolarized than −60 mV, input resistance of at least 5 MΩ and resting potentials that did not deviate by >10% for the duration of the recording. Data sets were rejected in which the stimulated nerve did not function fully throughout the recording, as determined by abrupt drops in EPSP amplitude. Data was acquired using an Axoclamp 900A amplifier, digitized using a Digidata 1440A and controlled using pClamp 10.3 software (Molecular Devices, Sunnyvale, CA). Electrophysiological sweeps were sampled at a rate of 10 kHz and filtered at 400 Hz. Data were analysed using MiniAnalysis (Synaptosoft), SigmaPlot (Systat Software) and Microsoft Excel. Average EPSP amplitude was corrected using nonlinear summation. FM1-43 dye labelling FM1-43 dye labelling using third-instar larvae was performed as described previously [54] . Briefly, larval preps were incubated with 4 μM FM1-43 dye (Invitrogen) in modified HL-3 containing 60 mM KCl for 5 min, and then washed with calcium-free saline. Images were captured using Zeiss LSM5 confocal microscope with a × 40 water-dipping objective. Fluorescence intensities were calculated using Image J and were normalized to the average labelling fluorescence intensity in controls. The ratio of unloaded/loaded was calculated by subtracting the fluorescence intensity remaining after unloading from the intensity of FM1-43 loading, and then divided by loaded fluorescence intensity: ( F loaded − F unload )/ F loaded . Drug treatment For proINDY drug treatment, dissected larvae with intact motor nerves were incubated in Schneider’s medium containing 0.2% dimethyl sulphoxide (vehicle control) or indicated concentrations of proINDY (with 0.2% dimethyl sulphoxide) for 30 min. Nerves were cut following incubation and were then used for staining, FM1-43 labelling or electrophysiological recording as described in the presence of proINDY or vehicle control. Western blotting Drosophila adult head extract was obtained by homogenizing adult heads collected on dry ice in high EDTA RIPA buffer (50 mM Tris–HCl, pH 7.5, 1% NP-40, 0.5% NaDoc, 150 mM NaCl, 0.1% SDS, 10 mM EDTA, 50 mM NaF, 1 mM Na 3 VO 4 , 250 nM cyclosporin A, protease inhibitor cocktail (Roche) and phosphatase inhibitor cocktail 1 (Sigma) using mortar and pestle. 10–20 μg protein homogenate was separated by SDS–PAGE and transferred to nitrocellulose membranes. Primary antibodies were diluted in blocking solution as following: rabbit anti-p-Synj, 1:5,000; guinea pig anti-Endo(GP60), 1:200; rabbit anti-Dap160, 1:5,000; rabbit anti-Mnb, 1:500, rabbit anti-Synj-1-rabbit. 1:200; mouse anti-dynamin, 1:200; mouse anti-complex V, 1:10,000 (MitoSciences); rabbit anti-phosphothreonine, 1:200; and rabbit anti-phosphoserine, 1:200 (EMD Millipore). To detect the amount of protein loading, nitrocellulose membrane was stained with Direct Blue 71. All values were normalized to control done within the same experimental set. Intensity of each band was quantified using Image J. Full images of key western blots are shown in Supplementary Fig. 7 . Quantitative RT–PCR One microgram of total RNA from adult fly brain was isolated using TRIzol reagent (Invitrogen), converted to complementary DNA using SuperScriptII reverse transcriptase (Invitrogen), and then used for quantitative RT–PCR with SYBR Green reagent (Applied Biosystems). Primers were designed from mRNA sequence to detect the indicated isoforms using PrimerExpress software v1.0 (Applied Biosystems). Primers specific for mnb-F: 5′-GTTGTACGATACTCA AGTTTGTG-3′ and 5′-CTGCTGGCATCATTTGAATTTG-3′. For mnb-H/E isoforms: 5′-CACCAAC GCAGCAGCAC-3′ and 5′-GACTAATCAGTAAGAACCGCAGG-3′. For mnb-G/I isoforms: 5′-AATGTCACGACGATCGCC-3′ and 5′-AGAGAGATACAGAGGCGTG-3′. For mnb-H/I isoforms: 5′-CCCTGGTTTATTGGCAGTC-3′ and 5′-TCGACCCGATCTCTATCTC-3′. Owing to sequence similarities between isoforms, primers specific for an individual isoform was not possible, except for mnb-F. Thermocycling was conducted in the ABI 7000 sequence detection system (Applied Biosystems) according to the manufacturer’s protocol. Sequence Detection System Version 1.7 software (Applied Biosystems) was used to analyse amplification plots. The relative quantity of amplified cDNA corresponding to each gene was calculated by using the ΔΔ C t method and normalized for expression of gapdh in each sample. Immunoprecipitation Flies were collected and frozen on dry ice and fly heads were isolated by passing through molecular sieves. Head protein extracts were obtained by homogenization as for western blotting. Protein homogenate (1.5 mg) was incubated with 1–5 μl antibody against specific proteins at 4 °C overnight. Protein complexes were precipitated by incubating with protein A/G PLUS-Agarose beads (Santa Cruz Biotechnology) at 4 °C for 2 h. The beads were washed with PBS four times and protein complexes were eluted by SDS–PAGE sample buffer. Phosphoprotein separation Isolation of phosphorylated and non-phosphorylated proteins was achieved using the PhosphoProtein Purification Kit (Qiagen) according to the manufacturer’s instructions. To ensure complete isolation of phospho- and non-phosphorylated proteins, 1.5 mg of protein homogenate was passed through two PhosphoProtein purification columns per genotype. Efficiency of phosphoprotein isolation was confirmed via western blottings using antibodies against phospho-serine and phospho-threonine by loading 10 μg of protein per lane. The level of phosphorylated proteins was determined by western blottings using antibodies against specific proteins in the phosphorylation-enriched and non-phosphorylation-enriched fractions normalized to the total protein level in the input. Protein purification His-tagged Mnb (His-Mnb) and His and HA doubly tagged Synj (His-Synj-HA) were obtained by cloning the Mnb-F and Synj-HA sequences from the pINDY6 vectors (used for transgenic fly generation) into pET15b vector (Novagen). BL21(DE3) competent E.coli. strain containing the expression plasmids were grown at 37 °C until A600 of the culture reached 0.6–0.8. Expression of the proteins was induced by the addition of isopropyl β- D -thiogalactopyranoside to a final concentration of 1.0 mM. After growth at 30 °C for 4 h, cells were harvested and stored at −80 °C until purification. For Mnb purification, His-Mnb was purified and eluted using the Ni-NTA Purification System (Invitrogen). Eluted His-Mnb was dialysed into kinase buffer (20 mM HEPES, pH 7.4, 10 mM MgCl 2 , 1 mM dithiothreitol (DTT) and 2 mM Na 3 VO 4 ) using Slide-A-Lyzer Dialysis (ThermoScientific). For Synj purification, isopropyl β- D -thiogalactopyranoside-induced bacterial cell lysate was incubated with anti-HA-agarose beads (Sigma Aldrich) at 4 °C overnight and washed with PBS for four times. To purify Synj from flies, adult head extract was prepared from flies overexpressing Synj-HA in neurons as described for immunoprecipitation. Extract was then incubated with anti-HA-agarose beads (Sigma Aldrich) at 4 °C overnight and wash with PBS. Mass spectrometry His-Synj or His-Synj PRD was purified as described above and separated by SDS–PAGE and stained with Coomassie blue. Purified Synj was then excised, denatured and reduced with DTT, alkylated with iodoacetamide and digested with trypsin [70] . Samples were analysed using an liquid chromatography/mass spectrometry system consisting of an Eksigent NanoLC Ultra 2D (Dublin, CA) and Thermo Fisher Scientific LTQ Orbitrap XL. Proteome Discoverer 1.4 (Thermo Fisher Scientific) was used for protein identification using Sequest algorithms. The following criteria were followed. For tandem mass spectrometry spectra, variable modifications were selected to include N,Q deamination, M oxidation and C carbamidomethylation with a maximum of four modifications. Searches were conducted against Uniprot or in-house customer database. Oxidized methionines and phosphorylation of tyrosine, serine and threonine were set as variable modifications. For the proteolytic enzyme up to two missed cleavages were allowed. Up to two missed cleavages were allowed for protease digestion and peptide had to be fully tryptic. MS1 tolerance was 10 p.p.m. and MS2 tolerance was set at 0.8 Da. Peptides reported via search engine were accepted only if they met the false discovery rate of 1%. There is no fixed cutoff score threshold, but instead spectra are accepted until the 1% false discovery rate rate is reached. Only peptides with a minimum of six amino acid lengths were considered for identification. We also validated the identifications by manual inspection of the mass spectra. In vitro dephosphorylation and re-phosphrylation of Synj Purified Synj-coupled to HA agarose beads (0.5 μg) was dephosphorylated by incubating with 5 units of AP (CIP) in NEBuffer 3 (New England BioLabs) at 37 °C for 1 h. Dephosphorylated Synj-coupled to HA agarose beads was then washed with PBS four times to remove CIP. For Mnb rephosphorylation, samples were subsequently treated with purified Mnb (0.5 μg) in kinase buffer (20 mM HEPES, pH 7.4, 10 mM MgCl 2 , 1 mM DTT and 2 mM Na 3 VO 4 ) at 37 °C for 1 h and then washed with PBS for four times to remove Mnb. Phosphatidylinositol 5′-phosphatase activity in vitro Phosphotidylinositol 5′-phosphatase activity was determined using either fly head extracts or purified Synj-coupled to HA agarose beads. Adult fly heads were homogenized in a buffer containing 10 mM HEPES, pH 7.4, 100 mM NaCl, 2 mM EGTA, 1% NP-40, 1 mM Na 3 VO 4 , 50 mM NaF, 250 nM cyclosporin A and protease inhibitor cocktail (Roche). One microgram of protein extract was used per assay. Alternatively, 0.5 μg of purified Synj coupled to HA agarose beads was used. Protein extract or purified Synj was incubated with labeled PI(4,5)P 2 (GloPIPs BODIPY FL-PI(4,5)P2, Echelon) in inositol phosphatase activity assay buffer (30 mM HEPES, pH 7.4, 100 mM KCl, 10 mM EGTA and 2 mM MgCl 2 ) at room temperature for 10–15 min or at 37 °C for 5–10 min. BODIPY-FL PI 4 P and BPDIPY-FL PI(4,5)P 2 were also spotted in separate lanes as standards. Lipid products were separated by TLC and visualized under ultraviolet radiation. Densitometry analyses were done using Image J. Synj was also eluted by adding SDS–PAGE sample buffer and Synj level was determined by western blottings. Phosphotidylinositol 5-phosphatase activity was normalized to the level of Synj. In vitro Synj interaction with endocytotic proteins Wild-type fly head extracts were obtained as for immunoprecipitation and incubated with 0.5 μg of purified Synj-HA coupled to agarose beads at 4 °C overnight. The protein complexes were then washed with PBS and eluted in SDS–PAGE sample buffer. Interactions were analysed via western blottings using antibodies against specific endocytotic proteins. Larval locomotor assay Deficits in larval locomotor behaviour were assessed similar to that described previously [54] . Briefly, larvae were washed with PBS and placed in 60-mm petri dish filled with 1% agarose. Using a moistened paint brush, third-instar larvae were collected and allowed to habituate until observation of progressive movement (~45 s). The number 0.5 cm 2 boxes entered was counted for a 30-s period. Synapse activity stimulation by High K + For NMJ immunochemistry, third instar larvae were dissected in HL-3 solution without Ca 2+ (110 mM NaCl, 5 mM KCl, 10 mM NaHCO 3 , 5 mM HEPES, 30 mM sucrose, 5 mM trehalose, 10 mM MgCl 2 , pH 7.2). High K + stimulation was achieved by replacing the solution with 90 mM KCl in HL-3 solution with Ca 2+ (25 mM NaCl, 90 mM KCl, 10 mM NaHCO 3 , 5 mM HEPES, 30 mM sucrose, 5 mM trehalose, 10 mM MgCl 2 , 1.5 mM CaCl 2 , pH 7.2) for 30 s. The samples were immediately fixed in 4% paraformaldehyde for 25 min and labelled with specific antibodies as for immunochemistry described previously. Pearson’s correlation coefficient for colocalization of Mnb with other proteins was determined using the Colocalization plugin in Image J. Percent increase in p-Synj was calculated by subtracting normalized p-Synj level of unstimulated synapse from normalized stimulated synapse (p-Synj/Synj-1 stimulate –p-Synj unstimulate /Synj-1 unstimulate ) × 100 For in vitro phosphatidylinositol 5′-phosphatase activity, third instar larvae were stimulated by incubating in 90 mM KCl in HL-3 solution with Ca 2+ for 5 min and immediately homogenized in inositol phosphatase activity assay buffer (30 mM HEPES, pH 7.4, 100 mM KCl, 10 mM EGTA and 2 mM MgCl 2 ). Phosphatidylinositol 5′-phosphatase activity was determined as described previously. The difference in phosphatidylinositol 5′-phosphatase activity was calculated by subtracting the PI4P/PI(4,5)P 2 ratio of unstimulated larvae from stimulated larvae. Statistics For paired samples, two-tailed Student’s t -test was used. For multiple samples, analysis of variance test followed by Bonferroni post-hoc test was used to determine statistical significance. All sample are biological replicates rather than technical replicates. Samples were randomized during dissection, image collection and data analyses to minimize bias. How to cite this article: Chen, C.-K. et al . Activity-dependent facilitation of Synaptojanin and synaptic vesicle recycling by the Minibrain kinase. Nat. Commun. 5:4246 doi: 10.1038/ncomms5246 (2014).